Design of synthetic yeast promoters via tuning of nucleosome architecture Model-based design of biological parts is a critical goal of synthetic biology, especially for eukaryotes. Here we demonstrate that nucleosome architecture can have a role in defining yeast promoter activity and utilize a computationally-guided approach that can enable both the redesign of endogenous promoter sequences and the de novo design of synthetic promoters. Initially, we use our approach to reprogram native promoters for increased expression and evaluate their performance in various genetic contexts. Increases in expression ranging from 1.5- to nearly 6-fold in a plasmid-based system and up to 16-fold in a genomic context were obtained. Next, we demonstrate that, in a single design cycle, it is possible to create functional, purely synthetic yeast promoters that achieve substantial expression levels (within the top sixth percentile among native yeast promoters). In doing so, this work establishes a unique DNA-level specification of promoter activity and demonstrates predictive design of synthetic parts. Synthetic biology design is ultimately constrained by our capacity to specify function of synthetic parts at the DNA sequence level. This capacity would redirect the field away from relying on a ‘parts-off-the-shelf’ strategy and toward an approach marked by pure, synthetic design and customizable specification. Toward this end, great strides have been made to enable model-based design of cellular behaviour [1] and to allow for rational design of small sequences (such as ribosome binding sites, transcription factors and enhancers) [2] , [3] , [4] , [5] , [6] , [7] , [8] . Yet, pure de novo design of full promoters, one of the most fundamental components in synthetic circuits, remains difficult, especially in eukaryotic model organisms like yeast. Traditional approaches spanning the last decade of promoter engineering efforts [8] rely upon part-mining [9] , mutagenesis strategies [10] , [11] , [12] and/or chimeric design [6] , [7] to identify promoter variants. More recently, data-driven rules have been developed to describe promoters as a first step toward comprehensive models [13] . In contrast, here we present the first approach for DNA-level specification of promoter activity on the basis of predicted nucleosome affinity. Previous studies have demonstrated both the importance of chromatin structure in promoter strength [14] as well as the capacity to alter transcription rates by modifying nucleosome binding sequences [13] . Following these studies, our overall hypothesis is that promoter activity can be predicted and controlled based on nucleosome architecture ( Fig. 1 ). To test this hypothesis, we made use of a previously-developed hidden Markov model to de novo predict nucleosome occupancy along an arbitrary DNA sequence [15] . This hidden Markov model has been validated in another study [15] and was found to be predictive of nucleosome position. By coupling this developed model along with our hypothesis, our approach can enable both the redesign of endogenous promoter sequences as well as the de novo design of synthetic promoters in a single design cycle. 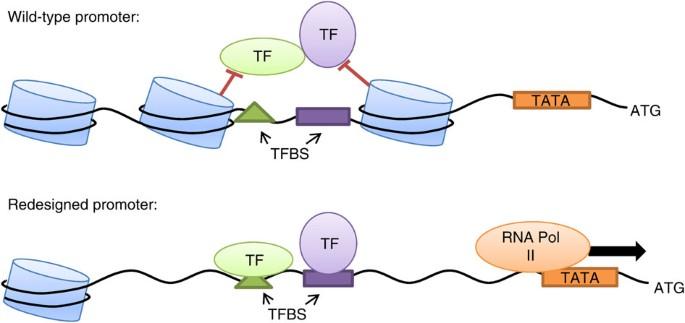Figure 1: A model for promoter strength. Native promoters can be redesigned for increased strength by decreasing nucleosome affinity. Transcription factors are designated ‘TF’ and binding sites are ‘TFBS’. Figure 1: A model for promoter strength. Native promoters can be redesigned for increased strength by decreasing nucleosome affinity. Transcription factors are designated ‘TF’ and binding sites are ‘TFBS’. Full size image Rational redesign of native yeast promoters Our earliest efforts in yeast promoter engineering [10] , [11] relied upon large-scale mutagenesis and selection to generate a TEF1 promoter library. This process clearly demonstrated that distributed point mutations in promoters can alter expression levels—although in most cases, lower expression than wild-type is obtained. Here, we sought to extract a design principle from this 15-member promoter library that collectively spans a 15-fold dynamic range in expression and encompasses between 5 and 71 mutations across 401 base pairs. By evaluating predicted nucleosome affinity across the 15-member TEF1 promoter library, we found that the cumulative sum of predicted nucleosome affinity across the entire promoter (hereafter referred to as the ‘cumulative affinity score’) is inversely proportional to promoter strength in a very robust, predictable manner, despite the great diversity of sequence and transcription factor binding site mutations ( Fig. 2a,b ). This strong correlation underpins the potential for nucleosome architecture to be used generically as a design principle for promoter engineering in yeast. 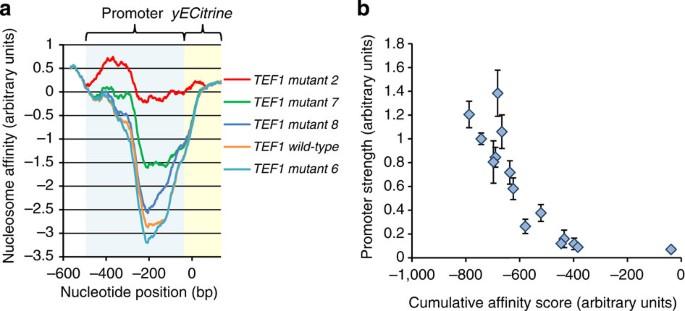Figure 2: Nucleosome affinity correlates to mutant promoter strength. (a) Computational nucleosome affinity profiles generated using a hidden Markov model15for severalTEF1mutant promoters10,11, withTEF1 mutant 2being the weakest andTEF1 mutant 6the strongest. (b) Experimental promoter strength as a function of cumulative affinity scores based on profiles inafor theTEF1mutant promoter library. Figure 2: Nucleosome affinity correlates to mutant promoter strength. ( a ) Computational nucleosome affinity profiles generated using a hidden Markov model [15] for several TEF1 mutant promoters [10] , [11] , with TEF1 mutant 2 being the weakest and TEF1 mutant 6 the strongest. ( b ) Experimental promoter strength as a function of cumulative affinity scores based on profiles in a for the TEF1 mutant promoter library. Full size image Using these results along with a computational exploration of sequence space, we established a framework to specify increased promoter strength at the DNA level by designing sequences with decreased predicted nucleosome affinity. Although this study focused on predictive increases in promoter activity, this approach may also be used more generally to decrease or otherwise tune promoter strength. Our nucleosome affinity minimization technique employed a greedy algorithm to minimize the cumulative affinity score over several rounds of optimization; in each round, all possible candidates differing by a single base pair were computationally generated and the candidate with the smallest cumulative affinity score was used as an input for the next round. Importantly, this optimization was bounded by the sequence-based requirement to avoid the destruction or creation of well-known transcription factor binding sites [16] , [17] ( Supplementary Software ). A greedy algorithm was chosen for computational convenience rather than for exhaustive nucleosome occupancy optimization. Moreover, we have validated this choice by finding that optimizing over all pairs of nucleotide substitutions in each round resulted in promoters with only slightly lower predicted nucleosome affinity although at a substantially increased computational cost (700 s per mutation versus 218,000 s per pair of mutations in the case of CYC1 ; Supplementary Fig. 1 ). Thus, the greedy algorithm is well-suited for the rapid identification of designer promoter sequences. As each round of the greedy algorithm evaluated all candidates differing by single base pair changes (a space on the order of 10 3 for each promoter tested), and because our design cycle consisted of 50–100 rounds, this proof-of-concept demonstration corresponds to sequence space searches of upwards of 10 5 in a facile manner. It should be emphasized that the searched space is small compared with the total available sequence space for a promoter of this length (10 156 ). The greedy algorithm chosen in this work is one way in which to computationally parse this large sequence landscape. The scope of this sequence space for the first round of the CYC1 promoter optimization is depicted in Fig. 3 . This initial search illustrates hot-spots in sequence space that result in lower cumulative nucleosome affinity scores. For example, in Fig. 3a , there are a series of variants clustered near the −100 base pair position that show decreased cumulative nucleosome affinity scores when mutated to T, and higher scores when mutated to G or C. Furthermore, it should be noted there are examples where changing a particular nucleotide to an A or T does not result in the lowest predicted score for that position even though AT-rich regions are generally less likely to bind nucleosomes. 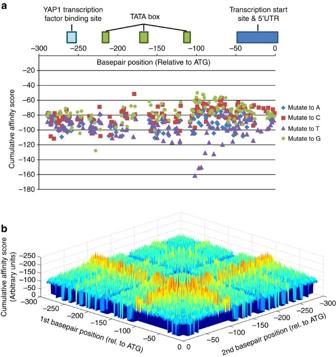Figure 3: Computational candidates generated for one round of the CYC1 promoter redesign. Each candidate queried for theCYC1promoter redesign was plotted for the first round of (a) a greedy algorithm searching over all possible single base pair changes per round and (b) a greedy algorithm searching over all possible double base pair changes per round. For the algorithm searching over all single base pair changes, known transcription factor binding sites, TATA boxes and transcription start sites are annotated. For the algorithm searching over all pairs, each point on the surface represents the most favourable pair of mutations (out of 16 possibilities) for a particular pair of positions. rel., relative. Figure 3: Computational candidates generated for one round of the CYC1 promoter redesign. Each candidate queried for the CYC1 promoter redesign was plotted for the first round of ( a ) a greedy algorithm searching over all possible single base pair changes per round and ( b ) a greedy algorithm searching over all possible double base pair changes per round. For the algorithm searching over all single base pair changes, known transcription factor binding sites, TATA boxes and transcription start sites are annotated. For the algorithm searching over all pairs, each point on the surface represents the most favourable pair of mutations (out of 16 possibilities) for a particular pair of positions. rel., relative. Full size image Using this approach, we successfully defined promoter sequences that experimentally increased the strength of four different native yeast promoters ( CYC1 , HIS5 , HXT7 and TEF1 ) that natively span an order of magnitude in expression level ( Fig. 4a , Supplementary Figs 2–7 compare wild-type promoter strengths and predicted nucleosome affinity profiles). In each of these cases, we used our approach to computationally redesign sequences for higher strength promoter variants by choosing the products of select rounds of optimization to synthesize, and then experimentally demonstrating improved transcriptional activity in a plasmid-based system. Furthermore, using the CYC1 promoter as a test case, we showed that a variety of expression levels can be generated by synthesizing the products of varying rounds of optimization, with CYC1v1 the product of an early round and CYC1v3 the product of a late round ( Supplementary Table 1 contains full promoter sequences). The greatest improvement in strength over wild-type for all of the redesigned promoters was 3.2-fold, exhibited by the CYC1v3 promoter, which is the result of the 30th round of optimization. Subsequent measurement of transcript level using quantitative PCR confirmed that the redesigned promoters increased transcriptional expression over each corresponding wild-type promoter ( Fig. 4b ). 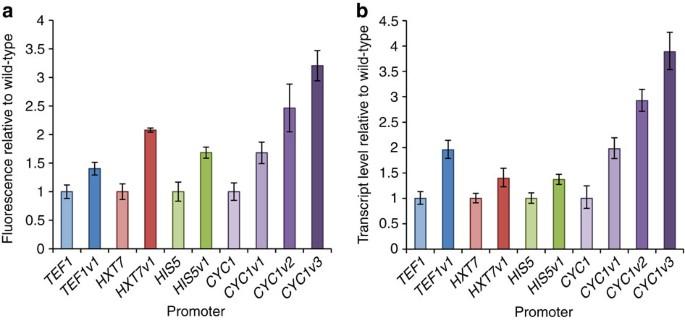Figure 4: Redesign of native yeast promoters for increased expression by decreasing nucleosome affinity. (a) Computationally redesigned promoters exhibiting upwards of 3.2-fold increases in fluorescence over wild-type. Error bars represent standard deviation from three biological replicates. SeeSupplementary Figs 2–7for a comparison of wild-type promoter strengths and predicted nucleosome affinity profiles. (b) Relative transcript level as measured by quantitative PCR for the promoters shown ina. Error bars represent s.d. from three technical replicates. Figure 4: Redesign of native yeast promoters for increased expression by decreasing nucleosome affinity. ( a ) Computationally redesigned promoters exhibiting upwards of 3.2-fold increases in fluorescence over wild-type. Error bars represent standard deviation from three biological replicates. See Supplementary Figs 2–7 for a comparison of wild-type promoter strengths and predicted nucleosome affinity profiles. ( b ) Relative transcript level as measured by quantitative PCR for the promoters shown in a . Error bars represent s.d. from three technical replicates. Full size image It should be noted that nucleosome architecture did not appear to be as limiting among the absolute strongest native promoters in yeast (including TDH3 and GAL1 ). While our previous work has demonstrated that these promoters have the capacity for increased expression through the use of chimeric hybrid promoters [7] , no increase in expression was seen in this work ( Supplementary Fig. 8 ), indicating that nucleosome architecture is likely evolutionarily optimized for these promoters. These two promoters represented the only cases in which false positives were identified by this algorithm. However, a nucleosome architecture approach could still likely be used to tune down the expression of these highest strength promoters. To confirm the biological underpinning of this design algorithm, nucleosome occupancy was measured via micrococcal nuclease digestion and quantitative PCR tiling array. This experiment demonstrated that nucleosome occupancy was reduced in CYC1v3 relative to wild-type CYC1 , as predicted by the model ( Fig. 5 ). These results clearly demonstrate that actual nucleosome occupancy was reduced in the redesigned promoter ( Fig. 5a ). 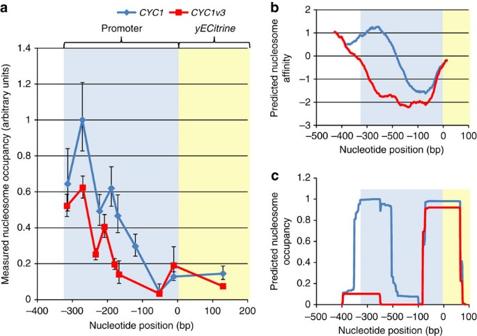Figure 5: Nucleosome occupancy is decreased in the CYC1v3 promoter relative to the CYC1 promoter. (a) Relative abundance of nucleosomal DNA as measured by micrococcal nuclease assays inCYC1andCYC1v3promoters. After micrococal nuclease digestion, copy number was measured across the promoter using a quantitative PCR (qPCR) tiling array. Each point represents the relative copy number of the qPCR amplicon centred at that base pair location. Relative copy number of each amplicon was calculated in comparison with a control amplicon in the ampicillin gene. Error bars represent s.d. from three technical measurements of each amplicon and ampicillin gene. The redesignedCYC1v3promoter exhibits lower nucleosome occupancy in the promoter region than the wild-type version. (b) Predicted nucleosome affinity profile for theCYC1andCYC1v3promoters using the hidden Markov model15. (c) Predicted nucleosome occupancy profiles for theCYC1andCYC1v3promoters using the hidden Markov model15. These results can be compared qualitatively with the computational predictions generated by the hidden Markov model, and complement previous work validating the predictive ability of the hidden Markov model [15] ( Fig 5b,c ). Collectively, these results confirmed our hypothesis that promoter strength may be controlled by manipulating nucleosome occupancy and demonstrated that nucleosome architecture can be used to specify sequence-function relationships for yeast promoters. Figure 5: Nucleosome occupancy is decreased in the CYC1v3 promoter relative to the CYC1 promoter. ( a ) Relative abundance of nucleosomal DNA as measured by micrococcal nuclease assays in CYC1 and CYC1v3 promoters. After micrococal nuclease digestion, copy number was measured across the promoter using a quantitative PCR (qPCR) tiling array. Each point represents the relative copy number of the qPCR amplicon centred at that base pair location. Relative copy number of each amplicon was calculated in comparison with a control amplicon in the ampicillin gene. Error bars represent s.d. from three technical measurements of each amplicon and ampicillin gene. The redesigned CYC1v3 promoter exhibits lower nucleosome occupancy in the promoter region than the wild-type version. ( b ) Predicted nucleosome affinity profile for the CYC1 and CYC1v3 promoters using the hidden Markov model [15] . ( c ) Predicted nucleosome occupancy profiles for the CYC1 and CYC1v3 promoters using the hidden Markov model [15] . Full size image Redesigned promoters function in multiple genetic contexts All of the above-described characterization was performed within a singular genetic context, namely a single plasmid design. Thus, we next sought to test the capacity for rationally designed promoters to function in alternative genetic contexts. Specifically, alternative contexts can be used to test the ability of the predicted changes to potentiate nucleosome architecture rearrangements independent of upstream and downstream DNA segments. Differences in the genetic contexts that surround the promoter, either due to the promoter’s location in the genome or due to the particular gene being expressed, could result in changes to the local chromosomal architecture and could therefore influence the final expression level of the promoter. This phenomenon of genetic loci-dependent expression is well-documented for the yeast genome [18] . First, the CYC1 series of redesigned promoters was evaluated with an alternative reporter gene. In this case, the yECitrine gene used in our previous experiments was replaced with a beta-galactosidase gene from Escherichia coli ( LacZ ). Beta-galactosidase activity was detected and the relative increase in expression level using this reporter was similar to that from the yECitrine constructs ( Fig. 6a ). In this case, CYC1v3 had a 3.8-fold higher relative expression compared with wild-type CYC1 . 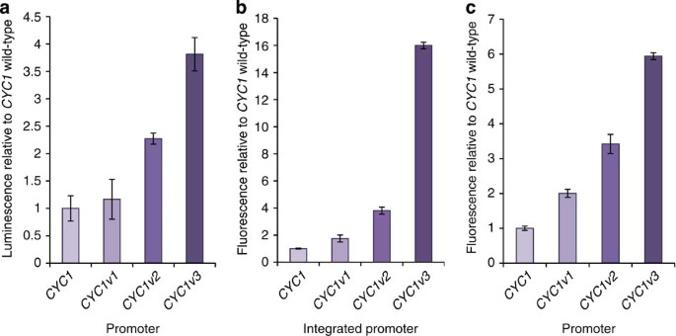Figure 6: CYC1 promoter redesigns have consistently increased expression levels in different genetic contexts. (a) Relative expression level from theCYC1promoter variants expressing the beta-galactosidase geneLacZas measured by a chemiluminescent assay. Background luminescence from a strain not expressingLacZwas negligible. (b) Relative expression level from theCYC1promoter variants expressingyECitrineand integrated into theTRP1locus of the BY4741 genome. (c) Relative expression level from theCYC1promoter variants expressingyECitrinewith theK. lactis URA3gene integrated upstream of the promoter. These plasmid constructs were the basis for the integration cassette used to create the strains measured in (b). Error bars represent s.d. from biological triplicate. Figure 6: CYC1 promoter redesigns have consistently increased expression levels in different genetic contexts. ( a ) Relative expression level from the CYC1 promoter variants expressing the beta-galactosidase gene LacZ as measured by a chemiluminescent assay. Background luminescence from a strain not expressing LacZ was negligible. ( b ) Relative expression level from the CYC1 promoter variants expressing yECitrine and integrated into the TRP1 locus of the BY4741 genome. ( c ) Relative expression level from the CYC1 promoter variants expressing yECitrine with the K. lactis URA3 gene integrated upstream of the promoter. These plasmid constructs were the basis for the integration cassette used to create the strains measured in ( b ). Error bars represent s.d. from biological triplicate. Full size image Second, the CYC1 series of redesigned promoters was evaluated in a genomic context. In this case, the Kluyveromyces lactis URA3 gene was cloned upstream of each CYC1 promoter variant as a marker gene, and the entire cassette was integrated into the TRP1 locus in the genome of Saccharomyces cerevisiae BY4741. Expression of yECitrine was measured using flow cytometry ( Fig. 6b ). The trend and rank order of increased expression level along this series was the same as for the plasmids (both for yECitrine and LacZ ). However, the relative fold-change in expression level was significantly higher for the integrated constructs than for the plasmids, with the highest increase from wild-type being 16-fold for CYC1v3 . To determine whether this difference was due to the move from the plasmid to the genome or due to the presence of the URA3 marker gene integrated upstream of the promoter, a set of plasmids containing the URA3 marker gene were also assayed for yECitrine expression ( Fig. 6c ). Interestingly, the fold-change in expression level for these constructs was intermediate between the original plasmid constructs and the integrated constructs, with the highest increase being 5.9-fold for CYC1v3 . It is therefore likely that both the addition of the marker gene and the integration of the cassette resulted in local repositioning of nucelosomes that changed the final ultimate nucleosome architecture of the expression cassette. Regardless, the redesigned promoters consistently increased expression level and maintained the same rank order, indicating that these rational changes are able to potentiate a decrease in the nucleosome occupancy of yeast promoters in a variety of genetic contexts, thereby increasing expression level in a general manner. Design and creation of synthetic yeast promoters As a second proof of concept, we sought to demonstrate that a model-guided approach can be used to create de novo promoters for synthetic biology without requiring the use of a native promoter as a scaffold. Previous attempts to create synthetic S. cerevisiae promoters usually relied upon hybrids of multiple promoter parts [7] , synthetic zinc finger transcription factor binding sites inserted into a scaffold of a native promoter [4] , [5] , the use of synthetic TALE transcription factors [19] or random libraries and screening [20] . A purely synthetic, de novo designed promoter created merely upon the arrangement of desired transcription factors has not been previously demonstrated. Specifically, our goal in this proof of concept was to demonstrate that, even without explicit information related to promoter architecture rules, it is possible to computationally specify active promoter sequences. To use our design and search strategy to create such a synthetic promoter, we specified two arrangements as initial lead scaffolds for the promoter design. Specifically, we utilized common glycolytic transcription factor binding sites embedded in random spacer sequences as the lead designs for our algorithm ( Fig. 7a , Supplementary Table 2 compares scaffolds to native promoters). This approach resulted in two synthetic base scaffolds: Psynth1 , and a shorter version Psynth2 , which were both used as inputs to our nucleosome affinity minimization technique. Three synthetic promoters were designed for Psynth1 and Psynth2 : one version from the sixth round of optimization, a second version from the 50 or 30th round and a third version from the 98 or 59th round, respectively. As a result, a total search space of 10 5 was evaluated over the entire design cycle for each base scaffold. The result was six DNA-specified promoters that were subsequently characterized. All six designs were found to be active promoters in vivo ( Fig. 7b ) that span nearly a 20-fold dynamic range with most of them being similar or higher in strength to the CYC1 promoter—a promoter representative of the mean expression level of native yeast promoters [21] . The power of our affinity minimization technique to increase promoter activity is especially evident in the case of Psynth1 . Psynth1v1 is only marginally higher in expression than the negative control, whereas Psynth1v2 is 3.5-fold higher and approaches the strength of CYC1 . Psynth1v3 is nearly 20-fold higher than Psynth1v1 and is on par with the strength of a commonly used promoter, the HXT7 promoter. Moreover, the substantial transcriptional capacity of this purely synthetic promoter places it in the sixth percentile of expression when compared with endogenous yeast promoters [21] . Furthermore, it should be noted that each of these synthetic promoters is quite distinct on a sequence level from native S. cerevisiae promoters. In fact, the most significant homology consisted of a 39 base pair sequence surrounding the TATA box of Psynth1 (E-value =0.48). Thus, our Psynth promoters are not enriched with native sequences and are therefore pure, de novo synthetic designs. Moreover, these de novo designed promoters did not require native spacing between transcription factors nor did they require the need to exactly mimic any given native promoter sequence as a scaffold. 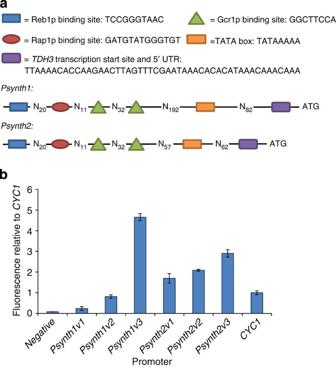Figure 7: Model-guided creation of de novo synthetic promoters. (a) Two synthetic lead sequences, each containing prescribed transcription factor binding sites and randomized linker sequences, were used forde novopromoter design. (b) Three computationally derived versions of each synthetic promoter were tested, one from an early round of optimization, one from an intermediate round and one from a late round.Psynth1v1andPsynth1v2are the result of the sixth round,Psynth1v2is from the 50th,Psynth1v3is from the 98th,Psynth2v2is from the 30th andPsynth2v3is from the 59th. Expression levels of the redesigned synthetic promoters spanned a nearly 20-fold range and all were functional. Error bars represent s.d. of three biological replicates. Figure 7: Model-guided creation of de novo synthetic promoters. ( a ) Two synthetic lead sequences, each containing prescribed transcription factor binding sites and randomized linker sequences, were used for de novo promoter design. ( b ) Three computationally derived versions of each synthetic promoter were tested, one from an early round of optimization, one from an intermediate round and one from a late round. Psynth1v1 and Psynth1v2 are the result of the sixth round, Psynth1v2 is from the 50th, Psynth1v3 is from the 98th, Psynth2v2 is from the 30th and Psynth2v3 is from the 59th. Expression levels of the redesigned synthetic promoters spanned a nearly 20-fold range and all were functional. Error bars represent s.d. of three biological replicates. Full size image Taken together, these results present the first DNA-level specification of promoter strength for yeast promoters on the basis of a nucleosome architecture model. We have demonstrated the potential of this approach for (1) the redesign of endogenous promoter scaffolds and (2) the design of de novo synthetic promoters. Specifically, native yeast promoters were redesigned into highly homologous sequences with promoter strengths up to 16-fold higher than their wild-type sequences. For each of the four promoter case studies, we improved activity by first interrogating ~\n10 5 promoter variants in silico (10 3 candidates were queried per round when searching over all possible single base pair changes, and 10 6 could be queried per round when searching over doubles, see Fig. 3 ), and then characterizing the products of selected rounds of the greedy algorithm in vivo . For the case of the CYC1 promoter, we chose the products of three different rounds of optimization to synthesize. This approach stands in stark contrast to the generation of large mutagenic libraries followed by screening. The extent of expression level increase did not always correlate with the absolute number of base pairs changed, as increases obtained in TEF1v1 required only five rounds of optimization ( Supplementary Table 1 contains full sequences). However, the utility of the greedy algorithm to sequentially identify increasingly optimal sequences was upheld for each case tested. Nevertheless, a more comprehensive, computational search of this sequence space may be used in place of the greedy algorithm to parse this complex landscape. Regardless, each of the redesigned promoters required multiple rounds (that is, base pair changes) to significantly increase expression, underscoring that these specific high-strength-potentiating combinations would be undetectable in random mutant libraries. In addition, we confirmed that these improvements were indeed due to decreased nucleosome occupancy in the case of the CYC1v3 promoter. Finally, we showed that these rationally designed promoters consistently display increased expression in a variety of genetic contexts, demonstrating that these directed changes are able to potentiate a decrease in nucleosome occupancy despite variation in the surrounding chromosomal architecture. Further, we created several fully synthetic yeast promoters which attain a variety of strengths and have minimal homology to any native sequence. The base promoter scaffolds for these synthetic promoters were only very loosely based on the native glycolytic promoters in yeast, demonstrating that close homology to native promoters may not be necessary for synthetic eukaryotic promoters. Given this surprising result, the range of synthetic promoter design possibilities is unbounded by traditional promoter architecture design rules inferred from native promoter structures. Furthermore, one of our synthetic promoters, Psynth1v3 , is on par with a commonly used promoter for metabolic engineering purposes, the HXT7 promoter, and resides among the top six percent of native yeast promoters with regard to strength [21] . This work confirms that nucleosome occupancy is an important causative factor limiting the strength of native yeast promoters and is likely an evolutionary mechanism for controlling transcriptional strength [22] . This method significantly advances the state-of-the-art in a field currently entrained in mutation and chimeric library construction by enabling the predictable specification of synthetic parts in single design-build-test cycles rather than by the generation of large libraries. Thus, this method opens the door to the rational design and creation of synthetic eukaryotic promoters as well as expands our capacity for pure synthetic biology design. Computational methods Nucleosome occupancy of native yeast promoters was optimized through the use of a computational algorithm. First, transcription factor binding sites present in the wild-type sequence were manually identified through the use of the Yeast Promoter Atlas [16] . Then, nucleotides outside these sites were systematically perturbed using a custom MATLAB script, which utilized a FORTRAN implementation of the Nucleosome Positioning Prediction (NuPoP) engine [15] to predict nucleosome affinity. Minor modifications to NuPoP were made to enable the acceptance of command-line inputs. The cumulative sum of nucleosome affinities over each candidate was then computed and the nucleotide substitution resulting in the largest decrease in total nucleosome affinity was saved as the product of one round of optimization. This sequence was then systematically perturbed as above so that successive increases in promoter strength were achieved in an iterative fashion. This MATLAB script additionally avoided the creation of new transcription factor binding sites [17] and also restricted promoter designs to those which could be synthesized as gBlocks by Integrated DNA Technologies, Inc. (Coralville, Iowa) which was the vendor chosen to provide the synthetic DNA in this project. The identity and placement of transcription factor binding sites in the synthetic promoter scaffolds were determined using a bioinformatics analysis of glycolytic promoters as a guide. The occurrence and relative positions of common transcription factor binding sites were catalogued and the average spacing values were calculated ( Supplementary Table 2 ). In addition to a consensus TATA box, four transcription factor binding sites were included in the upstream activating sequence area of the synthetic promoter: a Reb1p binding site, a Rap1p binding site and two Gcr1p binding sites. Consensus binding site sequences were used [17] . Psynth1 was designed using the average lengths between binding sites and Psynth2 was identical, except that the minimum length of the two longest regions (between the GCR1p binding site and the TATA box and between the TATA box and the transcription start site) was used instead of the average length in an attempt to make a shorter promoter. The TDH3 transcription start site and 5′ UTR was used for both synthetic promoters to prevent any confounding issues from having different 5′ UTR structures between promoters. Once the binding sites and relative positions were chosen, this information was then used as input to a custom MATLAB script to generate the Psynth series of vectors. First, the undetermined nucleotides between each transcription factor binding site were randomly seeded at a GC content of 35%. Once any inadvertent transcription factor binding sites generated in these regions were removed, nucleosome affinity was reduced in an iterative fashion as above. As before, the creation of new transcription factor binding sites or sequences which could not be synthesized was avoided. All computations were performed on an Intel Core 2 Duo processor running Windows 7. Strains and media S. cerevisiae strains BY4741 ( MAT a; his3 Δ 1; leu2 Δ 0; met15 Δ 0; ura3 Δ 0 ) and BY4741 Δ P CYC1 ( MAT a; his3 Δ 1; leu2 Δ 0; met15 Δ 0; ura3 Δ 0; P CYC1 ::ura3 ) were used in this study. BY4741 Δ P CYC1 was generated using the ‘delete and repeat’ knockout method [23] with the K. lactis URA3 gene from plasmid PUG72 as the selectable marker. Primers for the generation of the knockout cassette are in Supplementary Table 3 . Integration of the CYC1 promoter variants and yECitrine cassettes was completed by cloning the K. lactis URA3 gene upstream of each CYC1 promoter variant cassette (see below for plasmid construction) and then using the ‘delete and repeat’ method to integrate both genes into the TRP1 locus. See Supplementary Table 3 for primers. Yeast strains were propagated at 30 °C in yeast complete synthetic medium (CSM). CSM is composed of 6.7 g l −1 yeast nitrogen base, 20 g l −1 glucose and either CSM-HIS or CSM-URA supplement (MP Biomedicals, Solon, OH), depending on the required auxotrophic selection. E. coli strain DH10B was used for all cloning and plasmid propagation. DH10B was grown at 37 °C in Luria-Bertani (LB) media supplemented with 50 μg ml −1 of ampicillin. All strains were cultivated with 225 r.p.m. orbital shaking. Yeast and bacterial strains were stored at −80 °C in 15% glycerol. Plasmid construction All plasmids used in this study were based on the p413 yeast shuttle vectors [24] . These plasmids contain the HIS3 gene as the auxotrophic marker. The TEF1 and CYC1 promoters were available in the parent plasmid set. The TEF1 mutant series of promoters and the yECitrine and LacZ genes were cloned via PCR from plasmids [10] , [11] , [23] , [25] . The HXT7 and HIS5 promoters were cloned via PCR from extracted BY4741 gDNA obtained using the Wizard Genomic DNA Extraction Kit from Promega (Madison, WI). Redesigned and synthetic promoters were ordered as gBlock fragments from Integrated DNA Technologies, Inc. (Coralville, IA) and then cloned via PCR ( Supplementary Table 1 for promoter sequences and Supplementary Table 3 for all primer sequences). Standard cloning and bacterial transformations were performed according to Sambrook and Russell [26] . PCR reactions used Phusion High-Fidelity DNA Polymerase from New England Biolabs (Ipswich, MA) and followed supplier instructions; primers were purchased from Integrated DNA Technologies. Antarctic phosphatase and all restriction enzymes were purchased from New England Biolabs. Fermentas T4 DNA ligase and all other enzymes and chemicals were purchased through Thermo Fisher Scientific (Waltham, MA). Vectors were isolated using the Zyppy Plasmid Miniprep kit from Zymo Research Corp. (Irvine, CA) and DNA purification was performed with a Qiaquick PCR Cleanup kit (Qiagen, Valencia, CA). Plasmids were transformed using the EZ Yeast Transformation II Kit from Zymo Research Corp. according to manufacturer’s instructions. Flow cytometry Fluorescence from strains expressing the yECitrine gene was measured using a FACS Fortessa (BD Biosciences) in biological triplicate. Cells were grown for 16 h to mid-log phase from a starting OD 600 =0.005. For each strain, 10,000 events were collected using a YFP fluorochrome with a voltage of 355. Day-to-day voltage variability was mitigated by measuring all comparable strains on the same day. FlowJo (Tree Star Inc., Ashland, OR) was used to analyse data. For plasmids expressing yECitrine , positive YFP expression (as compared with strains expressing a control plasmid with no yECitrine ) was gated, and mean fluorescence values were calculated across the biological triplicates. For genome-integrated expression of yECitrine near autofluorescence values, mean fluorescence was calculated first, then the mean autofluorescence value (as measured from strains not expressing yECitrine ) was subtracted. Beta-galactosidase assay Strains expressing the LacZ gene were evaluated for beta-galactosidase activity through the chemiluminescent Gal-Screen system (Applied Biosystems). Yeast cultures were grown for 16 h to mid-log phase from a starting OD 600 =0.005. Before the assay, cultures were diluted with fresh media to approximately OD 600 =0.01–0.07. OD 600 was measured, and then cultures were treated with Gal-Screen Reaction Buffer according to the manufacturer’s instructions. Luminescence was quantified using a Mithras LB 940 luminometer (Berthold Technologies). Day-to-day variation was avoided by measuring all samples on the same day. The average luminescence across biological replicates was calculated. Quantitative PCR To measure mRNA levels resulting from redesigned promoters, quantitative PCR was performed. Yeast cultures were grown for 16 hours to mid-log phase from a starting OD 600 =0.005, and RNA was extracted using Zymolyase digestion of the yeast cell wall followed by the Quick-RNA MiniPrep kit according to manufacturer’s instructions (Zymo Research Corp.). cDNA was generated from the purified RNA via the High Capacity cDNA Reverse Transcription Kit (Applied Biosystems). Primers for qPCR were designed using the PrimerQuest tool and obtained from Integrated DNA Technologies ( Supplementary Table 3 for primers). Quantitative PCR was performed on a ViiA7 qPCR system (Life Technologies) using SYBR Green Master Mix from Roche (Penzberg, Germany), following the manufacturer’s instructions with an annealing temperature of 58 °C and 0.25 μl of cDNA product per 20 μl reaction. The ALG9 gene was used as a housekeeping gene, and the relative yECitrine transcript level was obtained by calculating the average values between three technical replicates for each sample. Nucleosome mapping Nucleosome position and density was mapped in the CYC1 and CYC1v3 promoters. The BY4741 Δ P CYC1 strain was used for this part of the study to prevent contaminating genomic sequence from confounding the results. Plasmids p413- CYC1 - yECitrine and p413- CYC1v3 - yECitrine were independently transformed into the strain as described above. Mono-nucleosome sized genomic DNA fragments were then isolated from each strain [27] . To conduct these measurements, 200 ml of culture was grown to approximately OD 600 =0.8. Cells were treated with 1% formaldehyde for 30 min at 30 °C. The reaction was stopped by adding glycine to a final concentration of 125 mM and cells were centrifuged at 3,000 g and washed twice in 20 ml of PBS. Cells were then resuspended in 20 ml Zymolyase buffer (1 M sorbitol, 50 mM Tris pH 7.4, 10 mM 2-mercaptoethanol), then spheroplasted with 50 U Zymolyase (Zymo Research Corp.) for 40 min at 30 °C. Cells were then washed once with 10 ml Zymolyase buffer and resuspended in 2 ml NP Buffer (1 M sorbitol, 50 mM NaCl, 10 mM Tris pH 7.4, 5 mM MgCl 2 , 0.075% NP 40, 1 mM 2-mercaptoethanol, 500 μM spermidine). Aliquots of 500 μl were split between four tubes for each sample, and CaCl 2 was added to a final concentration of 3 mM. Micrococcal nuclease (New England Biolabs) digestions were performed at concentrations ranging from 100–600 U ml −1 for 10 min at 37 °C. Reactions were stopped by adding 100 μl stop buffer (5% SDS, 500 mM EDTA). Proteinase K (New England Biolabs) was added to each tube at a final concentration of 100 mg ml −1 and incubated at 65 °C for approximately 8 h. DNA was purified using phenol-chloroform-isoamyl alcohol (25:24:1) extraction and ethanol precipitation. Resuspended DNA was treated with DNase-free RNase (Promega) for 30 min at 37 °C, then re-extracted using phenol-chloroform-isoamyl alcohol and ethanol precipitation. DNA was resuspended in 50 μl water and run in a 2% agarose gel. The dilution with the most apparent mono-nucleosome sized band (approximately 150 bp) was extracted using the Invitrogen Pure-Link gel extraction kit (Life Technologies, Carlsbad, CA). A tiling array of primer sets was designed for each promoter [14] to perform quantitative PCR. To accomplish this, primers were designed using the PrimerQuest tool and obtained from Integrated DNA Technologies ( Supplementary Table 4 for primers) and were placed approximately 50–100 base pairs apart. Quantitative PCR was performed as described above using 0.5 μl of mono-nucleosome DNA extract (at 10 ng μl −1 ) per 10 μl reaction. A section of the ampicillin gene on each plasmid was used as a control to account for any variation in total plasmid copy number between the two samples. Standard curves were created for each primer set using a serial dilution of the corresponding whole plasmid with concentration varying from 5 × 10 7 to 5 × 10 3 copies per μl. The relative copy number for each primer set in the promoter was calculated using these standard curves and comparing with the ampicillin primer set. How to cite this article: Curran, K. A. et al. Design of synthetic yeast promoters via tuning of nucleosome architecture. Nat. Commun. 5:4002 doi: 10.1038/ncomms5002 (2014).